Coherent topological transport on the surface of Bi2Se3 The two-dimensional surface of the three-dimensional topological insulator is in the symplectic universality class and should exhibit perfect weak antilocalization reflected in positive weak-field magneto-resistance. Previous studies in topological insulator thin films suffer from high level of bulk n -type doping making quantitative analysis of weak antilocalization difficult. Here we measure the magneto-resistance of bulk-insulating Bi 2 Se 3 thin films as a function of film thickness and gate-tuned carrier density. For thick samples, the magnitude of weak antilocalization indicates two decoupled (top and bottom) symplectic surfaces. On reducing thickness, we observe first a crossover to a single symplectic channel, indicating coherent coupling of top and bottom surfaces via interlayer tunnelling, and second, a complete suppression of weak antilocalization. The first crossover is governed by the ratio of phase coherence time to the inter-surface tunnelling time, and the second crossover occurs when the hybridization gap becomes comparable to the disorder strength. Weak localization (WL) and weak antilocalization (WAL) describe corrections to the classical electrical conductivity of two-dimensional (2D) electron gases due to coherent interference of time-reversed paths. The 2D surface state of the three-dimensional strong topological insulator (TI) is fundamentally distinct from other 2D electron systems [1] in that the Fermi arc encircles an odd number of Dirac points [2] , [3] , [4] , [5] , [6] , [7] , [8] . The TI surface is in the symplectic universality class and uniquely among 2D systems remains metallic and cannot be localized by (time-reversal symmetric) disorder [9] . In the absence of localization, the TI surface state is expected to exhibit perfect WAL described by, Hikami et al. [10] : where H 0 = ħ /4 Deτ φ is a characteristic field related to the phase coherence time τ φ and diffusion constant D , ψ is the digamma function, and α is the overall amplitude whose expected value for a single 2D channel is 1/2. However, WAL is sensitive to the competition between the phase coherence time τ φ and other time scales [11] ; in TI thin films, carriers may scatter into additional conducting channels (from top to bottom surface, or into the conducting bulk). Moreover, in finite-size samples inter-surface coupling can destroy the topological protection [12] , [13] , [14] , modifying the WAL behaviour. The question arises: at what size can a thin TI sample be treated as having decoupled topological surface states? In contrast to previous studies of WAL in TI thin films [15] , [16] , [17] , [18] , [19] , [20] , [21] , [22] where strong surface to bulk scattering dominates inter-channel coupling, here we report WAL measurements in gate-tuned, bulk-insulating Bi 2 Se 3 thin films where we expect negligible surface-bulk scattering. We find that the WAL behaviour in TI regime is governed by the ratio of τ φ to the inter-surface tunnelling time τ t = h /2Δ, where h is Planck’s constant and Δ is the hybridization gap induced by inter-surface tunnelling [12] , [14] . For thick films (17 nm), τ φ / τ t <1 and we observe the signature of a true 2D topological metal: perfect WAL according to equation (1) with α =½+½=1 corresponding to two decoupled TI surfaces each with α =½. A thickness and doping-dependent crossover is observed when τ φ / τ t >1 to a regime where α =½, indicating the coherent coupling of two TI surfaces. The result indicates that WAL is extraordinarily sensitive to sub-meV coupling between top and bottom topological surfaces, and the surfaces of a TI film may be coherently coupled even for thicknesses as large as 12 nm. For even thinner samples, Δ becomes comparable to the disorder strength and the Berry’s phase is completely randomized at low carrier density causing the suppression of WAL and WL, reflecting the loss of topological protection for strongly coupled surfaces. Characterization of Bi 2 Se 3 Hall bar devices We study mechanically exfoliated Bi 2 Se 3 single crystals [23] ranging in thickness from 5 to 17 quintuple layers (QL). 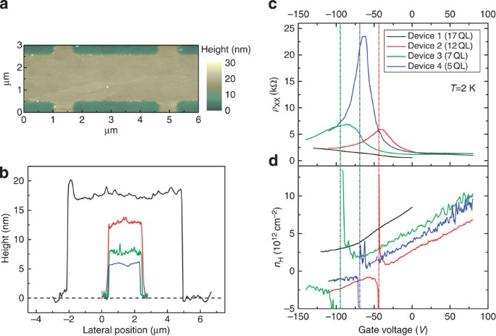Figure 1: Characterization of Bi2Se3Hall bar devices. (a) Atomic force microscopy image of 12 QL Bi2Se3Hall bar device. (b) Height profiles along width directions of the devices used in this study. (c) Longitudinal resistivityρxxand (d) sheet carrier densitynHdetermined from Hall measurement as a function of back gate voltage at the temperature of 2 K for 17 (black), 12 (red), 7 (green) and 5 (blue) QL devices. The dashed lines show charge neutrality points. Figure 1a shows a representative device (thickness 12 QL), where height profiles across the width direction of the 17, 12, 7 and 5 QL devices are shown in Fig. 1b . In order to achieve the topological transport regime, we employed molecular charge transfer p- type doping by thermal evaporation of 2,3,5,6-tetrafluoro-7,7,8,8-tetracyanoquinodimethane, described previously [24] (see also Methods, Supplementary Fig. S1 , and Supplementary Note 1 ). Figure 1: Characterization of Bi 2 Se 3 Hall bar devices. ( a ) Atomic force microscopy image of 12 QL Bi 2 Se 3 Hall bar device. ( b ) Height profiles along width directions of the devices used in this study. ( c ) Longitudinal resistivity ρ xx and ( d ) sheet carrier density n H determined from Hall measurement as a function of back gate voltage at the temperature of 2 K for 17 (black), 12 (red), 7 (green) and 5 (blue) QL devices. The dashed lines show charge neutrality points. Full size image Figure 1c show the longitudinal resistivity ρ xx and Hall carrier density n H =1/( eR H ) (where R H is the Hall coefficient, and e is the elementary charge) of the devices at a temperature of 2 K as a function of back gate voltage V g . We measure n H in the range of 2–7 × 10 12 cm −2 at zero gate voltage. The carrier density in the topological surface state at the bulk conduction band edge is ~0.8–1.0 × 10 13 cm −2 , hence the devices are close to the TI regime before application of a back gate voltage. Ambipolar electric field effects are indicated by the sharp peak of ρ xx ( V g ) and the sign change in n H at the charge neutrality points ( V g,0 , Fig. 1c dashed lines). The dependence of ρ xx ( V g,0 ) on temperature T in all of our devices, including 5 QL, shows metallic behaviour (see Supplementary Fig. S2 ), which is likely due to conduction through inhomogeneity-driven electron-hole puddles [24] , [25] . However, the thinnest (5 QL) device shows an anomalously large maximum ρ xx ( V g,0 ) of about 23 kΩ, which cannot be understood within the self-consistent theory for a Dirac band in the presence of charge disorder [24] , [26] , [27] , suggesting that the inter-surface hybridization gap Δ becomes important in determining the resistivity in this regime [12] . We note that true insulating behaviour (divergent ρ xx as T →0) is not observed for the 5 QL sample, but was previously observed for 3 QL Bi 2 Se 3 (ref. 13 ). More work is needed to understand the ρ xx maximum in the 5 QL sample (see Supplementary Note 2 for further discussion). WAL in the topological transport regime We now turn to discuss gate-tuned WAL behaviour in the TI regime. 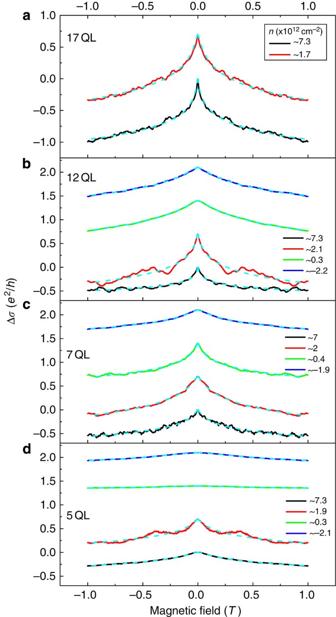Figure 2: WAL in the TI regime. Magneto-conductivity Δσas a function of perpendicular magnetic fieldHin (a), 17, (b), 12, (c), 7 and (d), 5 QL devices measured at 2 K at gate-induced carrier densities indicated in the legends. Dashed curves show least-square fits to equation (1). Zeros of all curves are offset by 0.7e2/hfor clarity. Figure 2 shows the magneto-conductivity Δ σ ( H ) for all four devices. Curves are taken at similar carrier density n = C g ( V g −V g,0 )/ e (where gate capacitance C g ≈11 nFcm −2 ) ranging from ≈7 × 10 12 cm −2 ( n- type) to −2 × 10 12 cm −2 ( p- type) except for the 17 QL device where only n- type carrier density (7 and 2 × 10 12 cm −2 ) could be observed due to relatively high initial doping. The data for the entire range of n and thickness can be fitted (dashed curves in Fig. 2 ) well with equation (1). The validity of equation (1) in the multichannel limit has been addressed in a number of previous studies [16] , [19] , [20] , [28] , finding that equation (1), in particular the logarithmic correction term, provides a robust physical description of WAL behaviour even in the multichannel limit irrespective of the Drude conductivity of each channel [20] , [28] . Therefore, α= m /2 probes the number of channels m . Moreover, although crossover to WL was predicted [29] in a gapped TI thin films (considered single 2D channel), further study of WAL in multi-channels including coherent coupling between channels [28] , as well as experimental observation in molecular beam epitaxy grown Bi 2 Se 3 (ref. 22 ) points out that WL can be neglected down to ~5 QL thickness. Our samples thus lie in the regime of dominant WAL. Figure 2: WAL in the TI regime. Magneto-conductivity Δ σ as a function of perpendicular magnetic field H in ( a ), 17, ( b ), 12, ( c ), 7 and ( d ), 5 QL devices measured at 2 K at gate-induced carrier densities indicated in the legends. Dashed curves show least-square fits to equation (1). Zeros of all curves are offset by 0.7 e 2 / h for clarity. 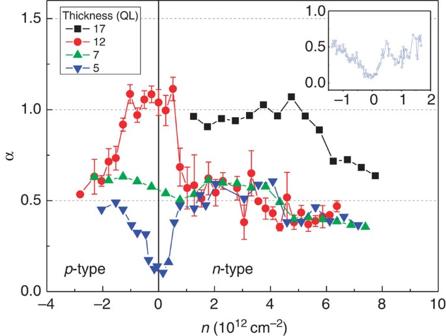Figure 3: Coupling of coherent transport in Bi2Se3surface states. Variation of the amplitude of WALαas a function of 2D carrier densitynfor 17 (black square), 12 (red circle), 7 (green triangle) and 5 QL (blue triangle) thick devices measured at 2 K. For the 12 QL device, the error bars show standard deviations determined from WAL measurements taken at five different thermal runs. The inset shows detailed behaviour of suppression of WAL for 5 QL at smalln. Full size image Coupling of coherent transport in Bi 2 Se 3 surface states Figure 3 shows the variation of α obtained from the fit to equation (1) as a function of n for 17 (black), 12 (red), 7 (green) and 5 (blue) QL devices measured at 2 K. In all devices α is close to 1/2 at high n ≈8 × 10 12 cm −2 , which we interpret as WAL in a single strongly coupled coherent channel [15] , [16] , [17] , [19] , [20] in the presence of surface to bulk scattering, as bulk states becomes energetically accessible (non-TI regime). Thus, we restrict the carrier density ranging n <6 × 10 12 cm −2 for investigating WAL behaviours in TI regime. The dependence of α on gate tuning shows very different behaviours depending on the thickness of the devices. The thickest device (17 QL) shows WAL consistent with two decoupled top and bottom topological surfaces ( α ≈1) starting at moderate n ≈6 × 10 12 cm −2 , maintained down to the minimum accessible n . Similar variation of α ranging from 0.7 to 1 was observed in Steinberg et al. [20] , with the application of top gate, and interpreted there as the decoupling of top surface and bulk (plus bottom) channels due to formation of band-bending-induced depletion layer. We do not rule out the possible contribution of bulk-surface scattering in 17 QL at high n. However, we note that this effect alone cannot explain the general behaviour of α for low n and thinner devices. Notably, we identify two crossovers in the 12 QL device: we observe sharp transition of α from ≈1/2 to ≈1 near n ≈1 × 10 12 cm −2 ( n- type), and back to 1/2 at n ≈−1 × 10 12 cm −2 ( p- type). Δ σ ( H ) in our devices include a moderate contribution from (universal) conductance fluctuations ( Fig. 2 ), as commonly observed in micro-fabricated Bi 2 Se 3 devices [16] , [21] ; the fluctuations are reduced by fitting to equation (1) over a large field range (0 T, 0.8 T). At the upper end of this field range, the magnetic length l B =( ħ / eH ) 1/2 becomes comparable to the electronic mean free path l mfp , approaching the regime where equation (1) may not be valid. However, we verified that the effect of increasing the field fitting range from (0 T, 0.02 T), where l B >> l mfp , to (0 T, 1 T), where l B l mfp , is only to reduce the fluctuations in α , without changing the average value, and that conductance fluctuations result in variation in α <0.1 in a given thermal run (see Supplementary Fig. S3c and Supplementary Note 3 ). Moreover, we repeated similar WAL measurements at 2 K for the 12 QL device on five different thermal runs, where the conductance fluctuation contribution is randomized, and find that the crossovers are reproducible within the experimental uncertainty represented by the standard deviation determined from the repetitive measurements ( Fig. 3 , error bars). This transition is absent in the 7 QL device, where WAL in the entire range of n indicates a strongly coupled single channel ( α ≈1/2). Finally, at an even smaller thickness (5 QL), we observe strong suppression of WAL for −1 × 10 12 cm −2 < n <1 × 10 12 cm −2 , (inset of Fig. 3 , see also Fig. 2d ). Figure 3: Coupling of coherent transport in Bi 2 Se 3 surface states. Variation of the amplitude of WAL α as a function of 2D carrier density n for 17 (black square), 12 (red circle), 7 (green triangle) and 5 QL (blue triangle) thick devices measured at 2 K. For the 12 QL device, the error bars show standard deviations determined from WAL measurements taken at five different thermal runs. The inset shows detailed behaviour of suppression of WAL for 5 QL at small n . Full size image Phase coherence time versus inter-surface tunnelling time We now examine the coherence time τ φ and compare with the estimated interlayer tunnel time τ t . We estimate τ φ = ħ /4 eDH 0 from the fits to equation (1) and using D=τ v F 2 /2 where Fermi velocity v F ≈3 × 10 7 cm s −1 for Bi 2 Se 3 (ref. 30 ), and the momentum relaxation time τ is calculated from the measured σ ( n ). τ t represents the characteristic time of transition (half the period Rabi oscillations) between localized states in two quantum wells with energy splitting Δ, thus τ t = h /2Δ. We estimate Δ in Bi 2 Se 3 by fitting the existing experimental data [12] to an exponentially decaying function. We estimated the range of Δ( t ) by including (1) sizable Δ in 2,3,4 and 5 QL (upper bound) and (2) all data from 2 to 8 QL (lower bound) in the fit and obtained Δ( t )=[992 meV] e −0.67[ t (nm)] and Δ( t )= [879 meV] e −0.62[ t (nm)] . The resultant range of Δ is 34.8–39.5, 9.1–11.44, 0.32–0.51 and 0.01–0.02 meV for 5, 7, 12 and 17 QL, respectively. (Theoretical calculations of finite-size effects in Bi 2 Se 3 predict systematically smaller Δ at a given thickness and also suggest that Δ shows oscillatory decaying behaviour [14] , which do not seem to be observed in the previous work [12] or this work.) 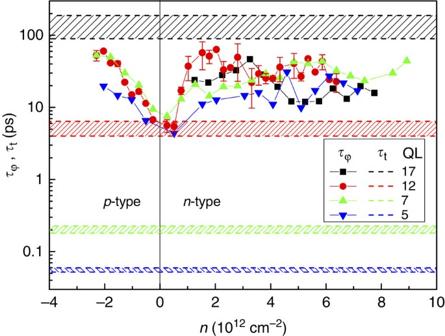Figure 4: Phase coherence time versus interlayer tunnelling time. Comparison of phase coherence time,τφ, determined from fit to equation (1) and transport scattering time to interlayer tunnelling time,τt, estimated from surface hybridization induced energy gap Δ as a function of 2D carrier densityn. Symbols are experimentally measuredτφfor 17 (black square), 12 (red circle), 7 (green triangle) and 5 QL (blue triangle) devices. The hatched areas with corresponding colours show estimated windows of inter-surface tunnelling timeτt. Figure 4 shows the estimated τ φ (symbols) and τ t (hatched areas) as functions of n for the different thickness samples. Upon gate tuning, τ φ changes by an order of magnitude ranging from ≈4 to ≈50 ps, and shows a sharp dip near n =0. For the 17 QL device, τ φ / τ t <1 in the entire range of n. In this limit, electrons on either surface lose coherence before scattering to the other, thus each surface acts as an independent coherent transport channel and α ≈1. In contrast, a crossover occurs from τ φ / τ t >>1 at high unipolar n - and p -type carrier densities to τ φ / τ t <1 near n =0 in the 12 QL device, which is consistent with the observed crossover from α =½ to α =1 ( Fig. 3 ). In the thinner device (7 QL), the condition τ φ / τ t >>1 is satisfied, and the two surfaces are strongly coupled ( α ≈1/2) for the entire range of n . The systematic tuning from coherent coupled to decoupled regimes upon variation of τ φ / τ t confirms that interlayer tunnelling is the primary coherent coupling mechanism in the TI regime. As τ t is primarily determined from the thickness of Bi 2 Se 3 thin films, whereas τ φ can vary significantly depending on the sample quality, we expect that the decoupling crossover thickness is not universal but can occur in different thickness if the surface phase coherence can be modified. For instance, decreasing phase coherence of the surface electrons by addition of magnetic impurities [31] should result in a reduced critical thickness above which decoupled coherent transport can be observed. In principle, temperature-dependent dephasing offers an additional opportunity to tune from coupled to decoupled surfaces. However, we observe weak dependence of the coherence time on temperature (see Supplementary Fig. S4 and Supplementary Note 4 ), which limits temperature as a parameter to control interlayer coherence. The weak temperature dependence of τ φ is observed elsewhere [21] but not understood, though it suggests an extrinsic mechanism. If the low-temperature decoherence can be improved, it may be possible to explore temperature-driven coherent coupling/decoupling of the TI surfaces. Figure 4: Phase coherence time versus interlayer tunnelling time. Comparison of phase coherence time, τ φ , determined from fit to equation (1) and transport scattering time to interlayer tunnelling time, τ t , estimated from surface hybridization induced energy gap Δ as a function of 2D carrier density n . Symbols are experimentally measured τ φ for 17 (black square), 12 (red circle), 7 (green triangle) and 5 QL (blue triangle) devices. The hatched areas with corresponding colours show estimated windows of inter-surface tunnelling time τ t . Full size image The behaviour described above is in general consistent in the 5 QL device except near the Dirac point, where WAL is strongly suppressed. The suppression of WAL can be understood in terms of the expected change of Berry phase θ B = π (1−Δ/2 E F ) in TIs [29] , [32] as a function of Δ and the Fermi energy E F ; θ B is reduced from π when hybridization induced gap opens. Assuming a gapped Dirac dispersion , we estimate E F ≤52 meV and θ B ≤0.67 π at | n |≤1 × 10 12 cm −2 . This range of n is comparable to the electron-hole puddle density n* ≈0.5 × 10 12 cm −2 per surface ( Fig. 1d ), hence transport occurs through a landscape of electron and hole puddles with θ B spanning the entire range 0≤ θ B ≤ π . It appears that in this regime of highly inhomogeneous Berry phase that both WAL and WL (expected as θ B →0) are suppressed. In contrast to semi-classical Boltzmann transport in Bi 2 Se 3 TI films, where the signature of finite-size effect appear only in the ultrathin limit (≤ 3 QL) (ref. 13 ), phase coherent transport offers an exquisitely sensitive probe of the hybridization of top and bottom transport channels, detecting a gap Δ as small as 0.3 meV in the 12 QL TI film [12] , as well as destruction of topological protection in the few QL film. We note that similar suppression of WAL was recently observed in thin epitaxial Bi 2 Se 3 of varying thickness (and Δ) but fixed E F (ref. 22 ), and a competition between WAL and WL was observed in gated 4 QL epitaxial (Bi 0.57 Sb 0.43 ) 2 Te 3 (ref. 33 ). Our observation of the WAL by tuning both E F and Δ (thickness) allows us to identify the ratio of τ φ / τ t as the driver for the crossover between coupled and decoupled surfaces, and the ratio of Δ to disorder strength as the driver for the crossover to the regime of suppressed WAL/WL. We expect that our results are important in identifying the regimes of carrier density and film thickness in which effects related to topological coherent transport can be observed in thin TI films. Bi 2 Se 3 field effect transistor fabrication Low-doped (carrier density~10 17 cm −3 ) bulk Bi 2 Se 3 single crystals with bulk resistivity exceeding 2 mΩ cm −1 at 300 K were grown by melting high purity bismuth (6N) and selenium (5N) in sealed quartz ampoules [23] . Crystals were exfoliated with Scotch tape and deposited on doped Si covered with 300 nm SiO 2 . Thin Bi 2 Se 3 crystals with thickness ranging from 5 to 17 nm were identified by combined use of optical and atomic force microscopy. From the atomic force microscopy height profile of Bi 2 Se 3 thin flakes, atomically flat surfaces with height variation <1 QL were chosen as channel area. Electron beam lithography, thermal evaporation and liftoff techniques were used to make electrical contact (Cr/Au: 5/70 nm). For accurate determination of the geometric factor, thin films were patterned into Hall bar geometry (see Fig. 1a ) with typical aspect ratio ( L / W ) of about 2 and shortest length exceeding 2 μm using Ar plasma at a pressure of ~6.7 Pa (5 × 10 −2 Torr). Molecular charge transfer doping was done by thermal evaporation of ~10 nm of 2,3,5,6-tetrafluoro-7,7,8,8-tetracyanoquinodimethane organic molecules (Aldrich) on top of the fabricated samples [24] . Measurement Transport measurements were performed using standard four-probe ac methods with low frequency (<17 Hz) excitation currents (r.m.s. amplitude 100 nA) using Stanford Research Systems SR830 Lock in amplifiers and a commercial cryostat equipped with 9 T superconducting magnet. For the 12 QL device, five different WAL measurements as a function of gate voltage at 2 K were conducted, where the sample was warmed up to 300 K and exposed to air for a few hours between thermal runs. How to cite this article: Kim, D. et al. Coherent topological transport on the surface of Bi 2 Se 3 . Nat. Commun. 4:2040 doi: 10.1038/ncomms3040 (2013).